Heisenberg-limited sensitivity with decoherence-enhanced measurements Quantum-enhanced measurements use quantum mechanical effects to enhance the sensitivity of the measurement of classical quantities, such as the length of an optical cavity. The major goal is to beat the standard quantum limit (SQL), that is, an uncertainty of order , where N is the number of quantum resources (for example, the number of photons or atoms used), and to achieve a scaling 1/N, known as the Heisenberg limit. So far very few experiments have demonstrated an improvement over the SQL. The required quantum states are generally highly entangled, difficult to produce, and very prone to decoherence. Here, we show that Heisenberg-limited measurements can be achieved without the use of entangled states by coupling the quantum resources to a common environment that can be measured at least in part. The method is robust under decoherence, and in fact the parameter dependence of collective decoherence itself can be used to reach a 1/ N scaling. Quantum mechanical noise imposes fundamental limitations on any measurement. The best-known example is the Heisenberg uncertainty relation, which provides a lower bound on the product of fluctuations of two non-commuting quantized variables. But even a classical system parameter x can in general not be measured with arbitrary precision with a finite number of measurements due to the statistical nature of any quantum state. A lower bound on the uncertainty is given by the smallest δx such that two quantum states ρ ( x ) and ρ ( x + δx ) lead to statistically significant differences for an optimally chosen observable. A similar problem exists in classical statistical analysis, in which one wants to distinguish between two probability distributions P ( x ) and P ( x + δx ), and the celebrated Cramér–Rao bound sets an ultimate lower bound on the uncertainty of a measurement of x based on the distinguishability of P ( x ) and P ( x + δx ) (ref. 1 ). That analysis has been generalized to the quantum world [2] and has become known as 'quantum parameter estimation theory'. Recently, the theory was used to prove lower bounds on the smallest measurable δx for unitary time evolution. It was shown that if N replicas of the quantum system evolve independently and linearly, for an initially separable state no uncertainty smaller than can be achieved, that is, the standard quantum limit (SQL), no matter how sophisticated the measurement. If initially entangled states are allowed, a 1/ N scaling of the uncertainty is the ultimate lower bound under otherwise identical conditions [3] , [4] , [5] , [6] . The use of non-classical states of light for Heisenberg-limited interferometry, notably the use of squeezed states, was proposed theoretically already in 1981 (ref. 7 ). So-called NOON states have been investigated for super-resolution [8] , [9] , [10] . However, decoherence of these highly non-classical states has so far prevented reaching an uncertainty that scales as 1/ N for systems with N ≫ 1 (refs 11 , 12 ). In ref. 13 entanglement-free Heisenberg-limited sensitivity of a phase-shift measurement was reported for several hundred quantum resources by passing light many times through the phase shifter. Decoherence arises when a quantum system interacts with an environment with many uncontrolled degrees of freedom, such as the modes of the electromagnetic field, phonons in a solid or simply a measurement instrument [14] . Decoherence destroys quantum mechanical coherence, and has an important role in the transition from quantum to classical mechanics [15] . It becomes extremely fast for a mesoscopic or even macroscopic 'distance' between the components of a 'Schrödinger cat'-type superposition of quantum states. Universal power laws rule the scaling of the decoherence rates in this regime [16] , [17] . Only recently could the collapse be time-resolved in experiments with relatively small 'Schrödinger cat' states [18] , [19] . However, decoherence can depend very sensitively on the initial state and the coupling to the environment. Entire decoherence-free subspaces (DFSs) can exist if the coupling operators to the environment have degenerate eigenvalues [20] , [21] , [22] , [23] , [24] . We show below that a collective coupling that depends on a parameter x of N quantum systems S i to a common 'environment' R can be used to measure x with an uncertainty that scales as 1/ N with an initial product state of all subsystems. The method works whether R is entirely under our control, or a reservoir with many degrees of freedom to which we have only partly access, that is, a collective decoherence process of the S i , as long as we can measure an observable of the environment. Model Consider N quantum systems S i coupled to a common environment R . The hamiltonian of the total system has the form where H i is the hamiltonian of system S i , and for simplicity we take the S i as non-interacting. H R denotes the hamiltonian of R , which may be itself a composite quantum system. Hamiltonian (1) can be a model of decoherence (in which case R would be the ensemble of many degrees of freedom of a 'reservoir' to which we have only partial access), or H ( x ) can generate a unitary evolution if R and S ={ S 1 ,..., S N } are completely under our control. The sum over ν runs over an arbitrary number of operators for each subsystem S i and R , but R v can also mean operators on different subsystems of R if R is composite (for example, positions of harmonic oscillators modelling a heat bath). To have a generic name for R that encompasses these different situations, we will refer to R as the 'quantum bus'. The entire dependence on x is included in the coupling operators S i,v ( x ). With 'collective couplings' (and with 'collective decoherence' if R is a reservoir) we mean S i,v ( x ) which do not depend on i . The smallest uncertainty δx with which x can be measured is found from quantum parameter estimation theory [2] . If the state of a system is given by a density matrix ρ ( x ), the smallest achievable δx is given by where we allow for M repetitions of the same measurement in identically prepared states ρ ( x ), and d s 2 is a metric on the space of density operators. It is related to the Bures' metric d Bures ( ρ,ρ+ d ρ ), with d ρ = ρ′ ( x )d x , by d s =2d Bures ( ρ,ρ+ d ρ ). For pure states, the Bures distance reduces essentially to their overlap, [25] . If ρ ( x ) and ρ ( x )+d ρ are related through a unitary transformation with generator ĥ , , then [2] An operational definition of δx is given by where we see that δx corresponds to the quantum uncertainty of an observable A in state ρ ( x ), suitably translated by the slope of 〈 A 〉 x into a fluctuation of x . As usual, for any observable A , 〈Δ A 2 〉≡〈 A 2 〉−〈 A 〉 2 , and all expectation values are with respect to ρ ( x ). Inequality (2) holds for all possible measurements, and for M →∞ a measurement exists that saturates the bound [2] . Model (1) cannot be solved in all generality. However, if the interaction is sufficiently weak it can be treated in perturbation theory. As we start in an initial product state at t =0, we can then relate properties of the full model to the single-particle dynamics of all S i and R . We first establish the fundamental lower bound on δx with the help of quantum parameter estimation theory, and then calculate δx for a given measurement on R . Quantum parameter estimation theory We decompose H ( x )= H 0 + H I ( x ), H I ( x )=∑ i,v S i,v ( x ) ⊗ R v , and switch to the interaction picture with respect to H 0 , with wave function |ψ I ( x,t )〉=exp(i H 0 t )|ψ( x,t )〉, |ψ( x,t )〉=exp(−i H ( x ) t )|ψ 0 〉. In Methods, we show that the Bures distance between the two states ρ ( x )=|ψ( x,t )〉〈ψ I ( x,t )| and ρ ( x +d x )=|ψ I ( x +d x , t )〉〈ψ I ( x+ d x , t )| is given by where we have defined the correlation function for any two operators A , B in the state | ψ 〉, K | ψ 〉 ( A, B )=〈 ψ | AB | ψ 〉−〈 ψ | A | ψ 〉〈 ψ | B | ψ 〉, H I ( x, t )=exp(−+i H 0 t ) H I ( x ) exp(−i H 0 t ) is the interaction hamiltonian in the interaction picture, and H′ I ( x, t )=∂ H I ( x, t )/∂ x . Equation (5) generalizes (3), which is recovered if [ H′ ( x ), H ( x )]=0 and H I ( x ) t = xĥ . From (2), we have For identical and identically prepared systems S i , S i,v = S v and for all i , and an initial product state we find where the expectation values for operators of S i ( R ) are taken in states | ϕ 〉 (| ξ 〉). Together with equation (6), this proves the existence of a measurement on S and R that gives a 1/ N scaling of δx min for N ≫ 1 and an initial product state, provided Measuring the quantum bus We now use directly equation (4) for showing that the 1/ N scaling can be achieved with the measurement of almost any observable A on R alone. The expectation values in equation (4) are in general time-dependent. This implies a time-dependent minimal uncertainty as well which does, however, not affect the scaling with N . We evaluate 〈 A ( t )〉 and 〈Δ A 2 ( t )〉 again by using second order perturbation theory in the interaction. The general results for these expressions are cumbersome, but simplify considerably if we make the following two assumptions: (1) the initial state of R is an eigenstate of A , ; and (2) A commutes with H R . Both assumptions taken together imply that the quantum bus is prepared in a noiseless state at t =0 (〈Δ A 2 (0)〉=0). Under the above two assumptions, we find which can also be used to obtain 〈 A 2 ( t )〉 and 〈Δ A 2 ( t )〉. Equation (4) then leads to In the limit of N ≫ 1, the term quadratic in N in dominates, and we find a 1/ N scaling of δx , provided that the denominator does not vanish. It is enough to measure an observable of the quantum bus R alone, with all subsystems initially in a product state. Decoherence All derivations so far apply perfectly well if R is an environment with many degrees of freedom, which we cannot fully measure. Measuring an observable A on only a subset of these implies a non-unitary evolution of S . This establishes immediately that we can reach a 1/ N scaling of δx , if x parametrizes a collective decoherence process and if we can measure at least some part of the environment. The example of superradiance that we will work out below is of this type. However, one might also be interested in how the unitary evolution generated by the hamiltonian (1) is affected by additional independent decoherence of the components S i and R . For Markovian decoherence, such a situation is described by a master equation for the density matrix W ( t ) of S and R of the form where L 0 X =[ H 0 , X ], and are Liouvillians of the Lindblad–Kossakowski type [26] for R ( S ), with The free evolution ( H I =0) still factorizes, such that, essentially, all expectation values and correlation functions are replaced by expectation values with respect to the relevant mixed states (see equation (37) in Methods). The 1/ N scaling is therefore robust under individual decoherence of the components, an eventually increased prefactor not withstanding. This is corroborated by further exact results for a pure interaction with decoherence added to all S i or to R (see Supplementary Discussion ), and by the example of superradiance below. Measuring the length of a cavity As example of an application, we now show how to measure the relative change of length δL/L of a cavity with an uncertainty of order 1/ N with an initial product state of N quantum resources. We first consider unitary evolution. Let N two-level atoms or ions ( N even, ground and excited states |0〉 i , |1〉 i for atom i , i =1,..., N ) be localized in a cavity, and resonantly coupled with real coupling constants g i to a single electromagnetic (e.m.) mode of the cavity of frequency ω and annihilation operator a (see Fig. 1 ), interaction hamiltonian where Owing to the spatial dependence of the e.m. mode in resonance with the atoms, the g i depends on the position z i of the atoms along the cavity axis and on the length L of the cavity (the waist of the mode is taken to be much larger than the size of the atomic ensemble) where k z = πn z / L , ɛ 0 denotes the dielectric constant of vacuum, V=LA the mode volume (with an effective cross-section A ), ɛ the polarization vector of the mode, and d the vector of electric dipole transition matrix elements between the states |0〉 i and |1〉 i , taken identical for all atoms. 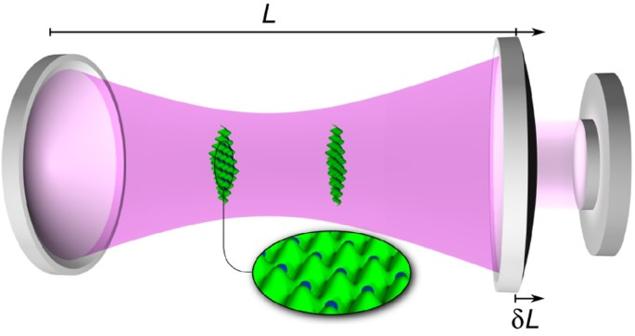Figure 1: Scheme for measuring the change of the length of an optical cavity. Natoms (or ions) are trapped at fixed positions in two two-dimensional optical lattices perpendicular to the cavity axis. A dipole transition of the atoms is in resonance with a single, leaky cavity mode. The atoms are initially prepared in a dark state in which destructive interference prevents the photons from being transferred from the atoms to the cavity mode. When the cavity lengthLchanges by a small amountδL, the true dark states evolve, and the initial state is exposed to collective decoherence, detectable by photons leaking out through the semi-reflecting mirror at a rate proportional toN2. This allows to measureδL/Lwith a Heisenberg-limited uncertainty of order 1/N, even if the initial dark state is a product state. Figure 1: Scheme for measuring the change of the length of an optical cavity. N atoms (or ions) are trapped at fixed positions in two two-dimensional optical lattices perpendicular to the cavity axis. A dipole transition of the atoms is in resonance with a single, leaky cavity mode. The atoms are initially prepared in a dark state in which destructive interference prevents the photons from being transferred from the atoms to the cavity mode. When the cavity length L changes by a small amount δL , the true dark states evolve, and the initial state is exposed to collective decoherence, detectable by photons leaking out through the semi-reflecting mirror at a rate proportional to N 2 . This allows to measure δL/L with a Heisenberg-limited uncertainty of order 1/ N , even if the initial dark state is a product state. Full size image If all g i are identical, we obtain the Tavis–Cummings model [27] . Here, we consider the situation where the atoms can be grouped into two sets with N /2 atoms each and coupling constants G 1 in the first set , and G 2 in the second set One way of obtaining two coupling constants may be to trap the atoms in two two-dimensional lattices perpendicular to the cavity axis (see Fig. 1 ). Note that it is not necessary to locate the atoms within a quarter wave-length of each other to obtain a DFS, as would be necessary without the cavity [28] . Distances which are integer multiples of the wave-length work just as well. In (15) we have neglected the transversal dependence of the mode, assuming that the atoms are localized at a distance from the cavity axis much smaller than the waist of the mode. However, this is for a computational convenience only. The initial product DFS states also exist if there is a radial variation of the g i , but describing the dynamics would become much more complicated as it would depend on all the different g i values. Assuming two different sets of coupling constants, the system is described by equation (1), where we identify a pair of atoms ( i,i+N /2) with subsystem S i , and the resonant cavity mode with the quantum bus R . The free hamiltonian H 0 consists of the energy of all atoms, , and the energy of the cavity mode, An expansion of the g i about L for a small change δL allows one to write the coupling in the form of (1) with and R 1 =a † , R 2 =a , and x ∝ δL / L (see Supplementary Information for the prefactor). For notational simplicity we restrict ourselves to the case where for x =0 the couplings are the same for the two sets, G 1 = G 2 = g , but this is by no means necessary for the method to work. A convenient basis for a pair of atoms is given by the 'singlet' and 'triplet' states with , , , and . As initial state of all S i and R we take the product state (7) with N→N /2, and , and for a cavity mode in the vacuum state. We obtain a time-independent , and from (6) which clearly scales as 1/ N for N ≫ 1. One might argue that a small amount of entanglement is present in | ϕ 〉, but the size of the cluster of atoms all entangled with each other (that is, a pair of atoms) is independent of N , such that it is legitimate to consider a pair of atoms as individual subsystem, and it is a product state of these subsystems that we consider. In Supplementary Information , we show that the product state can be prepared by letting the atoms interact pairwise. The initial state contains half a photon per atom. For a generic state the excitations stored in the atoms would start oscillating between the cavity mode and the atoms. However, for x =0 our initial state is a 'dark state', as destructive interference prevents the transfer of the photon from any pair of atoms to the cavity. When x deviates from zero, the perfect cancellation in the destructive interference is broken, and photons get transferred to the cavity. Measuring the number of photons constitutes an optimal measurement in the sense that the bound (16) is reached. To see this, we identify A = a † a in equation (13). This leads in a straightforward manner to which agrees with (16) for N ≫ 1, including the prefactor. After what was said in section 'Decoherence', it is clear that adding independent decoherence to all subsystems does not change the 1/ N scaling of δx min . We now show this explicitly by considering the situation of very strong damping of the cavity mode, the superradiant regime. The framework of section 'Decoherence' is suited for this analysis, but we adopt the well-developed theory of superradiance [29] , [30] , [31] , [32] to give an independent demonstration that δx min scales as 1/ N . Decoherence arises because of two processes: each atom can undergo spontaneous emission with rate Γ , because of its coupling to a continuum of additional e.m. modes. The damping of the cavity mode arises from the escape of photons with a rate 2 κ through one of the mirrors. In the notation of equation (14) and identification of a pair of atoms ( i,i + N /2) with S i , the generators Λ i and Λ R for these two processes read [29] , [30] , [31] , [32] Superradiance occurs in the overdamped regime where a photon transferred to the cavity leaves the cavity before it can feed itself back to the atoms, but induces emission in other atoms while in the cavity mode. Cavity decay is then the by far dominant process. We will therefore start by neglecting Γ, but treat spontaneous emission in Supplementary Information . The population of the cavity follows the occupation of the atoms adiabatically, and one can eliminate the cavity mode. This leads to the well-known and, for x =0, experimentally verified master equation of superradiance [29] , [30] , [31] , [32] , [33] , [34] for the reduced density matrix ρ s of the atoms in the interaction picture, The collective generators J ± are , The rate γ = g 2 / κ is independent of N . Collective decoherence is a two-stage process here, as photons stored in the atoms first need to be transferred to the cavity mode before they can leave the system. The dark states of section 'Measuring the length of a cavity' are therefore decoherence-free states. There is a large DFS containing DF states, including a 2 N /2 dimensional subspace in which the pair formed by the atoms l and l+N /2 can be in a superposition of | t − 〉 l and | s 〉 l [24] , [35] . A DFS of the same dimension also exists for non-identical couplings, but the coefficients in the linear combination of the singlet state need to be adapted accordingly, If after preparing the atoms in a DFS state corresponding to the initial couplings the length L of the cavity changes slightly, the coupling constants will evolve, , I =1, 2, and so will the DFS. Photons will leak out of the cavity as the original state becomes exposed to decoherence. There is a well-known connection between the photon statistics in the cavity mode and the excitation of the atoms, derived in ref. 30 for all couplings identical, One checks that this relation remains valid for small asymmetries x ≠0. Thus, instead of the number of photons in the cavity for a given value x one can calculate the excitation of the atoms, where, however, the observable itself becomes a function of x , For the initial product state (7) as considered above (with N → N p , , and ) we have from (19), Equation (20) is in principle valid only in the Markovian regime t ≫ 1/ κ , if is obtained from the solution of the Markovian superradiance master equation (19). However, the initial behaviour of is entirely determined by the value of at t =0, that is, the question of the Markovian approximation of the dynamics of does not arise, and equation (20) can therefore be used to calculate for short times up to order t 2 . From one finds immediately At this order κ does not intervene yet, as initially the cavity mode is in the vacuum state. The quadratic initial increase of 〈 n ph 〉 reflects the beginning of a Rabi oscillation between the excited atoms and the cavity mode. We expect this result therefore to be valid as long as Equation (23) agrees identically with the result one finds from the approach in section 'Decoherence' (see equation (37) in Methods). The fluctuations of n ph are obtained from Together with (20) one gets for with corrections of order ( g/κ ) 4 . From equations (4) and (23), we find which is identical to the minimal possible uncertainty, equation (16) for N ≫ 1. The validity of the short time expansions (21,22) is limited to Nγt ≪ 1, as can be seen from comparing the first order term with the zeroth order term. Inserting (21) in (20) gives therefore an analytical prediction of valid for in addition to the small-time result (23) for The agreement of based on (21) with the result from simulating (19) can be further improved by re-exponentiating according to before inserting it in (20). The limitation of validity of the small-time expansion does not pose a serious restriction in the bad cavity limit κ ≫ g , nor does it imply that the 1/ N scaling of the sensitivity breaks down beyond that regime. A full theoretical analysis for longer times will have to include the calculation of the superradiant propagator with broken SU (2) symmetry, however. For a non-Markovian description of superradiance is called for, which is beyond the scope of the present investigation. 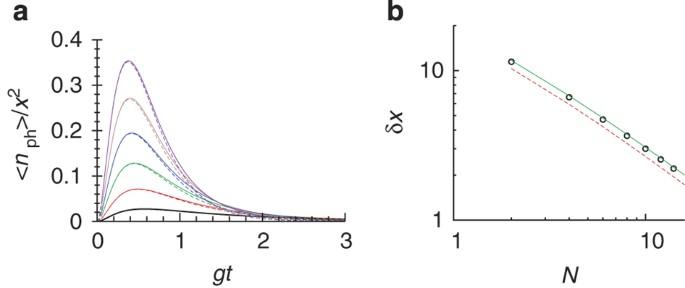Figure 2: Mean photon number and uncertaintyδxof the change of length of the cavity. (a) Mean photon number 〈nph〉 as a function of dimensionless timegt(wheregis the coupling constant of the atoms to the cavity mode) forN=2, 4, 6, 8, 10, 12 (black, red, green, blue, brown, violet), in units ofx2forx=0.1, and with photon escape rate from cavityκ=5g, obtained through numerical simulation of superradiance using a stochastic Schrödinger equation. The dashed lines with corresponding colours are analytical results valid up toNg2t/κ∼1 (see equations (20) and (21)). (b) Uncertaintyδx(see equation (4)) based onA=nphas function ofNforgt=0.0485 andx=0.01. Numerical results (circles) show the same 1/Nscaling as the ideal lower bound (red dashed line), equation (16), with slightly increased prefactor. Green continuous line is an analytical prediction based on an expansion of 〈nph(t)〉 for smallgt. Figure 2 shows that obtained numerically by simulating (19) through an equivalent stochastic Schrödinger equation, and integration of according to equation (20) agrees well with the result based on (21) for The stochastic Schrödinger equation for real ψ( t ) reads with and where d W ( t ) is a Wiener process with average zero and variance d t , and [26] . We used 2,000 equidistant time steps in the time interval t =0,..., 20/ g , 20 random realizations of the process for the simulation of 〈 n ph ( t )〉, and 400 realizations for the calculation of δx . Figure 2 also shows δx calculated from the numerical data for through equation (4), together with the fundamental lower bound δx min , equation (16). We see that at gt =0.0485, δx follows the optimal 1/ N scaling with only slightly increased prefactor. Figure 2: Mean photon number and uncertainty δx of the change of length of the cavity. ( a ) Mean photon number 〈 n ph 〉 as a function of dimensionless time gt (where g is the coupling constant of the atoms to the cavity mode) for N =2, 4, 6, 8, 10, 12 (black, red, green, blue, brown, violet), in units of x 2 for x =0.1, and with photon escape rate from cavity κ =5 g , obtained through numerical simulation of superradiance using a stochastic Schrödinger equation. The dashed lines with corresponding colours are analytical results valid up to Ng 2 t / κ ∼ 1 (see equations (20) and (21)). ( b ) Uncertainty δx (see equation (4)) based on A = n ph as function of N for gt =0.0485 and x =0.01. Numerical results (circles) show the same 1/ N scaling as the ideal lower bound (red dashed line), equation (16), with slightly increased prefactor. Green continuous line is an analytical prediction based on an expansion of 〈 n ph ( t )〉 for small gt . Full size image We emphasize that n ph allows to measure δL/L , not just to detect a change of L . Equations (20) and (21) relate 〈 n ph 〉 to x , and, unless the two lattices are situated at anti-nodes of the mode, the relation between and δL/L is linear to lowest order and independent of N : if we choose the position of the atoms such that we have Therefore, the measurement of 〈 n ph 〉 allows the measurement of δL/L . Several other practical questions, for example, the preparation of the initial state, and the robustness of the method with respect to fluctuations of the coupling constants, spontaneous emission and errors in the preparation of the initial state, are addressed in Supplementary Information . The superradiant regime has the advantage of providing direct access to the number of photons in the cavity. The average number of photons outside is simply obtained by integrating up to time t , as the photon escape rate is proportional to the average photon number inside the cavity [30] . The results for the scaling of δx with N based on A = a † a are therefore unaffected by detecting the photons that leave the cavity. Measuring the number of photons amounts to monitoring the decoherence dynamics, and we have thus an example where the parametric dependence of a collective decoherence process allows to achieve the Heisenberg limit with an initial product state. Our results may seem to conflict with the well-known theorem [4] that for unitary evolution of N independent quantum systems in an initial product state at best a scaling is possible. To see that there is no contradiction, it is helpful to consider the simple case where and H ( x ) commute, One then easily shows that to lowest order in d x , (with ħ=1) and are related by a unitary transformation with generator Let us furthermore restrict ourselves to a single operator per subsystem, that is, v =1 only, and to the linear x dependence S i ,1 ( x )= xS for all i , and R 1 = R . A few lines of calculation lead to for an initial product state, from equation (7). All expectation values of S in (25) are in state | ϕ 〉, those of R in the state | ξ 〉. Inserting (25) into (3) and (2), we find that for N ≫ 1 and that is, the Heisenberg limit can be achieved with an initial product state. Clearly, for the case considered above the unitary transformation generated by is not necessary to achieve the 1/ N scaling. We therefore simplify the reasoning further by considering the case H 0 =0. We are then left with a pure interaction, But this is not a hamiltonian of the form required by the theorem in ref. 4 . In our case all subsystems couple in a non-trivial manner to the common quantum bus R and are therefore not independent. This turns out to be the decisive difference. The SQL can be recovered for the standard situation of N independent subsystems through a R that acts only trivially on R , that is, R = 1 , such that This makes obvious the rather ironic fact that quantum fluctuations in R help and are necessary to achieve the 1/ N scaling. The prefactor of the 1/ N behaviour is smallest for an initial state with an equal weight superposition of the eigenstates of R pertaining to its largest and lowest eigenvalues r min and r max , in which case This simple example also allows to corroborate that to achieve the 1/ N scaling one need not measure the S i at all, and almost any measurement on R suffices. Consider an initial product state and for We then have Let A be an observable on R , which does not commute with R , that is, there are at least two eigenstates | r 0 〉 and | r 1 〉 such that It is sufficient to consider an initial state of R , which is a superposition of these two states, for example, we may take and an observable If all subsystems S i are prepared in the same state with s i =s , one finds and Inserted in equation (4) this leads to the exact result valid for all x . This shows that the 1/ N scaling can be reached by measuring almost any observable of R , as long as it does not commute with R . Furthermore, equation (27) allows a simple quantum-information theoretical explanation of the effect: The final state reflects the accumulated phase from the interaction of all the systems S i with the common quantum bus R . 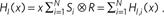Figure 3: Quantum circuit that reproduces the interaction hamiltonian. Nquantum systemsSiprepared all in the eigenstate |s〉 ofSi,Si|s〉=s|s〉 in equation (26), lead to a total accumulated relative phase between states of the quantum busRthat is proportional toxN. This allows a measurement ofxwith a precision that scales as 1/N, even though the initial state is a product state, by measuring any observableAonRalone that does not commute withR. Figure 3 shows an equivalent quantum circuit that reproduces state (27). One subsystem S i after another imprints the same phase on the components of the state of R . Equation (27) also makes obvious that a measurement of the S i alone does not allow to achieve the 1/ N scaling, as the state of R will collapse on a single state | r m 〉, and one only gets an irrelevant global phase. Thus, measuring the quantum bus is not only sufficient, but also necessary for the 1/ N scaling of δx . We also see that the measurement of is optimal if r 0 , r 1 correspond to the smallest and largest eigenvalues of R , respectively. Figure 3: Quantum circuit that reproduces the interaction hamiltonian . N quantum systems S i prepared all in the eigenstate | s 〉 of S i , S i | s 〉= s | s 〉 in equation (26), lead to a total accumulated relative phase between states of the quantum bus R that is proportional to xN . This allows a measurement of x with a precision that scales as 1/ N , even though the initial state is a product state, by measuring any observable A on R alone that does not commute with R . Full size image In ref. 13 , an adaptive measurement technique was demonstrated that allows one to achieve Heisenberg-limited uncertainty by using only an initial product state. The method is based on phase estimation [36] , but instead of using a NOON state of N photons, independent photons were passed N times through the same phase shifter. This amplifies the phase by a factor N , but it was shown that in the presence of losses the scaling of the sensitivity with N is at most improved by a constant factor [37] compared with the classical case for N →∞. A common feature of both phase estimation and our method is that a measurement is performed on a common quantum system that interacts with all other quantum systems. However, our method is more general. It incorporates decoherent and unitary evolutions in the same framework, and allows one to use collective decoherence as a signal. Second, phase estimation was developed for a multi-qubit system with controlled, sequentially turned on interactions, and an x -dependence in the free evolution. Hamiltonian (1) on the other hand can be used to describe substantially more complex systems, with possibly non-trivial dynamics in the absence of the collective interaction, and with interactions that do not commute with the Hamiltonians of the free constituents. Furthermore, the interaction is simultaneous such there is no bandwidth penalty in the accumulation of the phase, nor is there a need to re-sample a phase shift many times. Our method requires a collective interaction between N separable quantum systems and a common quantum bus, an initial noiseless state in the sense discussed above, and the possibility to measure at least part of the quantum bus. In the case of incomplete measurement of the quantum bus this implies the need of a collective decoherence process with a decoherence-free initial state. Besides atoms in a cavity one might consider circuit-QED systems [38] , trapped ions coupled to a common phonon mode [39] , or quantum dots coupled to micro-resonators [40] or to photonic crystals [41] . Both unitary evolution or a decoherence process can be useful, as long as the collective interaction between the N quantum resources and a common quantum bus depends on the parameter x to be measured. To summarize, we have developed a general theory of collectively enhanced quantum measurements based on the interaction of N quantum systems with a common 'quantum bus'. The latter can be a simple quantum system, or an environment with many degrees of freedom to which we have only partial access. We have shown that if the collective interactions depend on a parameter x , the Heisenberg limit (that is, a 1/ N scaling of the uncertainty of x ) can be reached with an initial product state, and by measuring almost any observable of the quantum bus. We have used quantum parameter estimation theory to establish that a 1/ N scaling of the uncertainty is indeed optimal in this setup. We have given a simple quantum-information theoretical interpretation of the effect, and we have analysed in detail a possible experimental implementation of the measurement of the change of the length of a cavity with an uncertainty that scales as 1/ N . The proposed measurement principle offers an attractive way out of the dilemma of ubiquitous decoherence that has so far plagued quantum-enhanced measurements. First of all, there is no need to build highly entangled states, which are extremely fragile under decoherence for large N . Simple product states will do, and decoherence of some parts of the system does not affect the 1/ N scaling of the minimal uncertainty. Second, parameter-dependent collective decoherence is covered itself by our new measurement principle. Indeed, decoherence is a process in which quantum interference effects can have an important role. This is exemplified by the very existence of DFS, and can lead to exquisite sensitivity when a DFS is disturbed. Instead of trying to suppress decoherence at all costs, one might therefore be better off exploiting its parametric dependence. Bures distance for unitary evolution The state vector in the interaction picture obeys the time-dependent Schrödinger equation with the interaction hamiltonian The general solution of (29) is given by where T denotes the time-ordering operator. To second order in the perturbation H I ( x,t ), the overlap between reads with all expectation values with respect to | ψψ 0 〉. We assume that the derivatives of H I ( x ) with respect to x are hermitian operators, in which case the term linear in d x is purely imaginary. The lowest order term in the squared overlap is then of order d x 2 . One finds in a straightforward manner the squared Bures distance (5). Decoherence of subsystems Markovian decoherence of the S i and R on top of the unitary evolution generated by H ( x ) can be described by equation (14). The single system dynamics (that is, all S i and R taken separately, L I =0), can be solved formally by exponentiating the Liouvillians. We will again treat L I ( x ) in perturbation theory. The density matrix W I ( t ) of S and R in the interaction picture is related to the one in the Schrödinger picture, W ( t ), by and obeys the master equation With equation (33) we have defined the free propagator , and is the interaction Liouvillian in the interaction picture. We decompose furthermore To second order in L I we have With an initial product state, we obtain the zeroth as all propagators are trace-preserving, and Similarly, by explicitly writing we obtain the first order term where . We generalize the second simplifying assumption in section 'Measuring the quantum bus' to and with some function f A ( t ) [30] . This implies that the initial state is decoherence-free concerning the decoherence of R alone. This is a natural assumption for the state of an environment initially in thermal equilibrium, or for a quantum bus in its ground state, such as an initially empty cavity mode (see the example of superradiance). We then have again 〈 A ( t )〉 1 =0. To second order in the interaction we find where The index k is arbitrary, k =1,..., N , as we have assumed all systems S k identical and identically prepared. All x -dependence is in the operators S v . Equation (37) also gives 〈 A 2 ( t )〉 by replacing A → A 2 , and 〈 A ( t )〉 2 to order O ( H I 2 ). The equation obtained by inserting these expressions into equation (4) generalizes the result (12) to decoherence on top of the unitary evolution considered in section 'Measuring the quantum bus'. We see that the basic structure of the result for δx , and in particular its scaling with N is unchanged, but the expectation values and correlation functions are replaced by more complicated expressions involving in general mixed states and non-unitary evolution of individual subsystems. Quantum parameter estimation for a Markovian master equation In standard descriptions of decoherence, one traces out the heat bath and gets a master equation for the reduced density matrix ρ s of S alone. Using quantum parameter estimation theory generalized to non-unitary evolution, we now show that for Markovian decoherence with an initially decoherence-free state, measuring an arbitrary x -independent observable on S alone gives at best a This corroborates the result found for unitary evolution that the important quantum system to measure is the common quantum bus R , rather than S . The Markovian master equation for ρ s ( t ) obtained by tracing out R has the Lindblad–Kossakowski form where we work in the interaction picture and assume that there is no additional unitary evolution. The F α ( x ) are arbitrary linear (not necessarily hermitian) operators, which have inherited the x -dependence from the interaction hamiltonian H I ( x ), and d is the total number of generators. Note that we can restrict ourselves to an initially pure state, as for any linear propagation one cannot do better with a mixed state than with the pure states from which it is mixed [42] . We expand the Markovian time evolution to first order in t , and linearize F α ( x ) about the value of x where we want to measure. We set that value, without restriction of generality, to zero, that is, F α ( x )= xF α ′ + F α (0), and assume that the initial state is decoherence-free at x =0. The Bures distance can still be evaluated in a straightforward manner as the state at x =0 remains pure. One finds As a consequence, the ultimate quantum limit of the sensitivity with which the parameter x can be estimated from the parametric dependence of the master equation, starting from a pure state | ψψ 〉, reads With we obtain For an initially entangled state, can be of order N 2 . This can be seen from the example of the GHZ state and a single generator with the Pauli z matrix for subsystem i . Then and one obtains a 1/ N scaling of δx min , just as in the case of unitary evolution. However, if the initial state factorizes, there are no correlations between different subsystems r and s , and we thus have only the sum of correlations in all subsystems, which is at most of order N , and δx min scales as again just as in the case of unitary evolution. This shows once more that a measurement of an x -independent observable on S does not allow to do better than in the standard situation of unitary evolution of S without coupling to a common quantum bus. Interestingly, superradiance is described by a master equation of S alone after tracing out the cavity mode. But a measurement on R (the number of photons in the cavity) translates in that case to a measurement on the S i that depends itself on x . In this way, it is still possible to achieve a 1/ N scaling of δx . How to cite this article: Braun, D. and Martin, J. Heisenberg-limited sensitivity with decoherence-enhanced measurements. Nat. Commun. 2:223 doi: 10.1038/ncomms1220 (2011).